Multimode optomechanical dynamics in a cavity with avoided crossings Cavity optomechanics offers powerful methods for controlling optical fields and mechanical motion. A number of proposals have predicted that this control can be extended considerably in devices where multiple cavity modes couple to each other via the motion of a single mechanical oscillator. Here we study the dynamic properties of such a multimode optomechanical device, in which the coupling between cavity modes results from mechanically induced avoided crossings in the cavity’s spectrum. Near the avoided crossings we find that the optical spring shows distinct features that arise from the interaction between cavity modes. Precisely at an avoided crossing, we show that the particular form of the optical spring provides a classical analogue of a quantum non-demolition measurement of the intracavity photon number. The mechanical oscillator’s Brownian motion, an important source of noise in these measurements, is minimized by operating the device at cryogenic temperature (500 mK). Optomechanical systems are typically modelled as a single cavity mode whose eigenfrequency depends linearly on the displacement of a mechanical oscillator [1] . This ‘single-mode’ model of optomechanics gives an accurate description of devices in which there is a clear separation of frequencies (for example, between the mechanical frequency and the cavity mode spacings), and when only a single cavity mode is strongly driven [2] . Single-mode optomechanical devices have been used to realize a number of goals in recent years, including demonstrations of quantum effects associated with Gaussian states of the cavity field and/or the mechanical oscillator [3] , [4] , [5] , [6] , [7] , [8] , [9] , [10] , [11] , [12] , [13] , [14] . For some optomechanical devices the single-mode description breaks down and more complex behaviour can occur. In particular, devices in which multiple cavity modes couple to each other via the oscillator’s motion are predicted to offer novel means for controlling and measuring both the mechanical motion and electromagnetic fields [15] , [16] , [17] , [18] , [19] , [20] , [21] , [22] , [23] . Such a mechanical coupling between the cavity modes can be produced by applying strong coherent drives to the modes (in which case adiabatic elimination of the mechanical degree of freedom results in an effective coupling between the drives’ sidebands) [22] , [23] . This approach can be realized in a very wide range of optomechanical systems, since most cavities possess several modes that can be driven strongly, and whose eigenfrequencies depend upon the oscillator’s displacement. Recent experiments have used this approach [24] , [25] (or a related approach that combines strong drives with a piezoelectric material [26] ) to transfer modulation sidebands between different wavelengths, including from microwave to near-infrared. A different method for mechanically coupling cavity modes (and one which does not require multiple strong drives) is to employ devices in which the cavity’s eigenmodes (rather than eigenfrequencies) depend strongly upon the oscillator’s displacement. This situation occurs when the oscillator’s displacement causes crossings in the cavity’s spectrum: these crossings are typically avoided (owing to broken symmetries within the device) [27] , [28] , [29] , and in the vicinity of each avoided crossing the cavity’s eigenbasis depends strongly upon the oscillator’s displacement [29] , [30] . Theoretical studies of the resulting coupling show that it can offer improved performance over single-mode devices, for example, in producing squeezed states of the mechanical oscillator and optical field [19] , [20] , [21] . Perhaps more importantly, the multimode coupling associated with avoided crossings offers capabilities that are fundamentally distinct from those of single-mode devices, with applications in macroscopic matter-wave interferometry [18] and measuring the phonon statistics of a driven mechanical oscillator [15] , [16] . Avoided crossings are not a generic feature in optomechanical systems, but have been demonstrated in devices based on the membrane-in-the-middle design [27] , [29] , [31] , [32] , ultracold atoms [33] and whispering gallery mode resonators [34] , [35] . To date, measurements of these systems have mostly focused on static spectroscopy of the cavity modes (that is, to determine the parameters of the avoided crossings) [27] , [28] , [29] , [31] , [32] , [33] , [34] , [35] . However the utility of the avoided crossings arises from their dynamical effects, which have received much more limited experimental study [33] , [34] , [35] . Here we address three outstanding issues related to multimode optomechanical devices based on cavities with avoided crossings. First, we describe thorough measurements of the optomechanical dynamics in the vicinity of the avoided crossings. Far from the crossings, we find a behaviour that is dominated by the conventional dynamical back action [1] of the laser driving the cavity; in contrast, near the crossings the behaviour is dominated by the elastic energy stored by the intracavity light. Second, we exploit the elasticity of the intracavity light at the crossings to demonstrate a classical analogue of a quantum non-demolition measurement of the cavity’s photon number. Third, the device is operated at temperature T =500 mK, which minimizes the impact of thermomechanical noise, and should aid in future work directed at observing quantum effects in multimode optomechanical systems. These results complement the earlier studies of classical multimode dynamics in different systems, for example, in purely mechanical devices [36] , [37] , purely electromagnetic devices [38] and devices in which multiple mechanical modes couple via a single electromagnetic mode [39] , [40] , [41] . Experimental setup The experimental setup is shown in Fig. 1a . It consists of a Si 3 N 4 membrane (1 mm × 1 mm × 50 nm) placed inside a Fabry–Perot optical cavity and cooled by a 3 He cryostat to T =500 mK. The cavity finesse F =4,000 (linewidth κ /2π=1 MHz), and the membrane’s fundamental mode resonates at ω m /2π=354.6 kHz with a quality factor Q= 100,000. Laser light with wavelength λ =1,064 nm enters the cryostat via an optical fibre. This light is coupled from the fibre to the cavity via cryogenic free-space optics that are aligned in situ using piezoelectric motors. Similar motors are used to adjust the membrane’s position, tip and tilt within the cavity. An additional piezoelectric element allows for fine displacement of the membrane along the cavity axis and for excitation of the membrane’s vibrational modes. 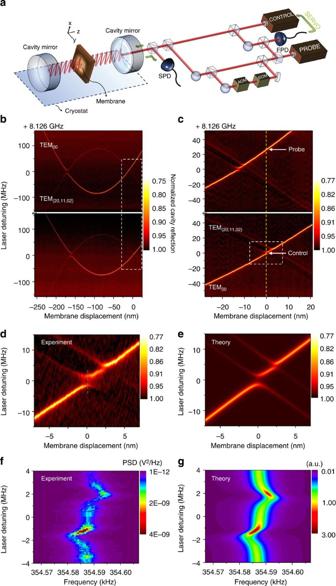Figure 1: System overview and cavity reflection spectroscopy. (a) Schematics of the cryogenic ‘membrane-in-the-middle’ setup. Two separate lasers (‘probe’ and ‘control’) address a Fabry–Perot cavity containing a Si3N4membrane atT~500 mK. Two modulators (AOM and EOM) in the probe beam path allow for Pound–Drever–Hall locking to the cavity and heterodyne detection of the membrane’s motion. (b) Cavity reflectivity, plotted as a function of the membrane’s static displacementzdisand laser detuning Δ. The upper and lower plots are measured by the probe and the control lasers, respectively. The cavity’s TEM00singlet mode and the TEM{20,11,02}triplet modes are visible. (c) A closer view of the dashed area inbshowing avoided crossings between the singlet and triplet modes. The crossings in the modes addressed by the probe beam occur roughly 10 nm away from the crossings in the modes addressed by the control beam. Atzdis=0 nm (dashed yellow line), the probe beam can be used to detect membrane motion while the control beam addresses the avoided crossings. (d) Zoom-in of the avoided crossings measured with the control beam. (e) The calculated cavity spectrum corresponding to the same parameters as ind. (f) Measured power spectral density of the membrane’s Brownian motion as a function of control laser detuning Δ (the range of Δ is given by the dashed green line ind). For this measurementzdis=0 nm andPin=80 μW. Shifts in the membrane’s resonance frequency, consistent with quadratic optomechanical coupling, are visible around the cavity resonances at Δ=±1.6 MHz. (g) Calculated power spectral density of the membrane’s Brownian motion for the same parameters as inf. Figure 1: System overview and cavity reflection spectroscopy. ( a ) Schematics of the cryogenic ‘membrane-in-the-middle’ setup. Two separate lasers (‘probe’ and ‘control’) address a Fabry–Perot cavity containing a Si 3 N 4 membrane at T ~500 mK. Two modulators (AOM and EOM) in the probe beam path allow for Pound–Drever–Hall locking to the cavity and heterodyne detection of the membrane’s motion. ( b ) Cavity reflectivity, plotted as a function of the membrane’s static displacement z dis and laser detuning Δ. The upper and lower plots are measured by the probe and the control lasers, respectively. The cavity’s TEM 00 singlet mode and the TEM {20,11,02} triplet modes are visible. ( c ) A closer view of the dashed area in b showing avoided crossings between the singlet and triplet modes. The crossings in the modes addressed by the probe beam occur roughly 10 nm away from the crossings in the modes addressed by the control beam. At z dis =0 nm (dashed yellow line), the probe beam can be used to detect membrane motion while the control beam addresses the avoided crossings. ( d ) Zoom-in of the avoided crossings measured with the control beam. ( e ) The calculated cavity spectrum corresponding to the same parameters as in d . ( f ) Measured power spectral density of the membrane’s Brownian motion as a function of control laser detuning Δ (the range of Δ is given by the dashed green line in d ). For this measurement z dis =0 nm and P in =80 μW. Shifts in the membrane’s resonance frequency, consistent with quadratic optomechanical coupling, are visible around the cavity resonances at Δ=±1.6 MHz. ( g ) Calculated power spectral density of the membrane’s Brownian motion for the same parameters as in f . Full size image Two lasers are used to address two cavity modes that are separated by 8.13 GHz (roughly twice the free spectral range). The first laser is the ‘probe’ beam; it is locked to the cavity and detects the membrane’s motion via a heterodyne scheme. The second laser is the ‘control’ beam, and is locked to the probe beam with a controllable frequency offset. This control beam produces the multimode optomechanical interactions that are the main focus of this paper. Additional information about the setup is provided in Supplementary Fig. 1 and the Supplementary Methods . Static spectroscopy Figure 1b and c show the cavity reflection spectra measured separately by the probe beam (upper plots) and the control beam (lower plots). In each case the reflection was recorded as a function of laser detuning and the membrane’s static displacement z dis . The brightest curve corresponds to the TEM 00 mode (‘singlet’), while the slightly dimmer curves correspond to the TEM {20,11,02} (‘triplet’) modes. The triplet modes are nearly degenerate, but can be resolved in the closer view shown in Fig. 1c . The longitudinal order of the singlet mode differs by one from that of the triplet modes; as a result their resonance frequencies ω cav undergo roughly opposite detuning as a function of z dis (ref. 28 ), and so appear to cross each other near z dis =0 nm and z dis =−160 nm. A closer view of the apparent crossing near z dis =0 nm shows that two of the triplet modes avoid the singlet mode ( Fig. 1d ) [29] . The optomechanical dynamics that occur near these avoided crossings is the main focus of this paper. Because the probe and control beams address modes with slightly different wavelength, the avoided crossings for the two beams occur at different values of z dis . This makes it possible to position the membrane so that the probe beam addresses a mode that is not a part of an avoided crossing (and so simply provides an efficient readout of the membrane’s oscillatory motion z osc ( t )) while the control beam addresses modes that undergo an avoided crossing (thereby producing multimode optomechanical coupling). Such a position is indicated in Fig. 1c as a dashed yellow line, which we define as z dis =0 nm. Optomechanical dynamics near the avoided crossings To demonstrate the impact of the avoided crossings on the membrane’s motion, we first position the membrane at z dis =0 nm where the detuning of the modes addressed by the control beam is quadratic to lowest order, that is, . In this case, each intracavity photon is predicted [27] , [42] to produce an optical spring that shifts ω m by an amount (the primes indicate differentiation with respect to z osc , and z ZP is the amplitude of the membrane’s zero-point motion). Figure 1f plots the power spectral density of the membrane’s Brownian motion (recorded by the probe beam) as the control beam’s detuning Δ is varied. These data show the two qualitative features of quadratic coupling. First, the change in the membrane’s resonance frequency δ ω m is proportional to the number of intracavity photons (that is, δ ω m (Δ) has even symmetry about each cavity resonance with an approximately Lorentzian shape). Second, the sign of δ ω m is set by the sign of (that is, positive when the laser is tuned to the higher-frequency cavity mode and negative when the laser is tuned to the lower-frequency mode). In contrast, for conventional single-mode optomechanics (in which the detuning is linear: ω cav ∝ z osc ) δ ω m (Δ) has odd symmetry about a cavity resonance and its sign is the same regardless of which cavity mode is excited by the laser [1] . To make a more quantitative comparison with the theory, we use multimode optomechanics theory [42] to calculate the cavity reflection, optical spring and optical damping in the presence of the avoided crossings (see the Supplementary Fig. 2 and the Supplementary Note 1 for more details). The majority of the parameters in this theory are determined by fitting the cavity’s static spectrum to expressions that include three cavity modes. Figure 1d,e shows a comparison of the measured and fitted reflection, and the Supplementary Table 1 lists the values of all the system parameters. To determine the remaining parameters, and to test the predictions of this model with respect to the dynamical behaviour, we measured the membrane’s Brownian motion at several values of z dis between −1 nm and +1.25 nm. At each value of z dis , the control beam detuning Δ was varied over a range that included both of the cavity modes participating in the avoided crossing. For each value of Δ, the membrane’s resonance frequency ω m and mechanical damping rate γ m were determined by fitting the Brownian motion spectrum. 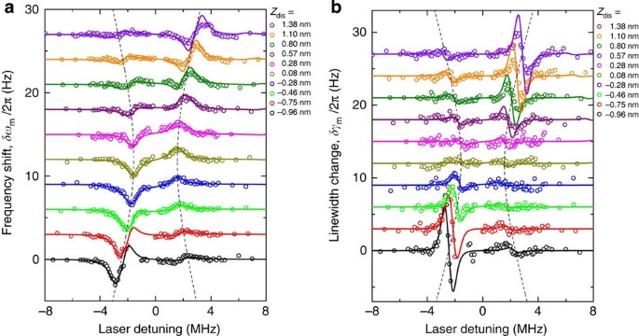Figure 2: Optomechanics near the cavity’s avoided crossings. (a–b) Changes in the frequency (a) and linewidth (b) of the membrane’s fundamental mode, plotted as a function of the control laser detuning Δ and the membrane’s static displacementzdis. The avoided crossing occurs atzdis=0 nm. The solid lines are the fits described in Methods and theSupplementary Note 2. The dashed lines indicate the cavity resonances. For clarity, each curve is shifted vertically by 3 Hz. For large negative values ofzdis, the lower-frequency cavity mode produces larger optomechanical effects than the higher-frequency cavity mode due to the fact that it corresponds to the TEM00mode, which is more strongly coupled to the driving laser (as can be seen inFig. 1d). For large positive values ofzdis, the situation is reversed. Figure 2 shows the changes in these quantities (that is, the optical spring δ ω m and the optical damping δ γ m ) as a function of Δ for each value of z dis . Figure 2: Optomechanics near the cavity’s avoided crossings. ( a – b ) Changes in the frequency ( a ) and linewidth ( b ) of the membrane’s fundamental mode, plotted as a function of the control laser detuning Δ and the membrane’s static displacement z dis . The avoided crossing occurs at z dis =0 nm. The solid lines are the fits described in Methods and the Supplementary Note 2 . The dashed lines indicate the cavity resonances. For clarity, each curve is shifted vertically by 3 Hz. For large negative values of z dis , the lower-frequency cavity mode produces larger optomechanical effects than the higher-frequency cavity mode due to the fact that it corresponds to the TEM 00 mode, which is more strongly coupled to the driving laser (as can be seen in Fig. 1d ). For large positive values of z dis , the situation is reversed. Full size image When the membrane is furthest from the avoided crossing (that is, for the uppermost and lowermost curves in Fig. 2 ), the features in δ ω m and δ γ m show odd symmetry about the cavity resonances (which are indicated by dashed lines), consistent with conventional single-mode optomechanics and linear coupling. As z dis approaches 0 nm, the features in δ ω m and δ γ m decrease in size, consistent with the decreasing slope of the cavity detuning near the avoided crossing. Precisely at the avoided crossing (olive-coloured data in Fig. 2 ), the odd-symmetry feature in δ ω m is completely absent and is replaced by an even-symmetry feature (as discussed above in the context of Fig. 1f ). The solid lines in Fig. 2 are calculated from the model described in Methods. These calculations use the parameters determined from the cavity’s static spectrum ( Fig. 1d,e ), as well as three additional fit parameters. A complete description of the fitting process is given in the Supplementary Figs 3–7 and the Supplementary Note 2 . The agreement between the data and the fits in Fig. 2 indicates that multimode optomechanics theory provides an accurate description of this system, particularly in the vicinity of multiple avoided crossings between the cavity modes. 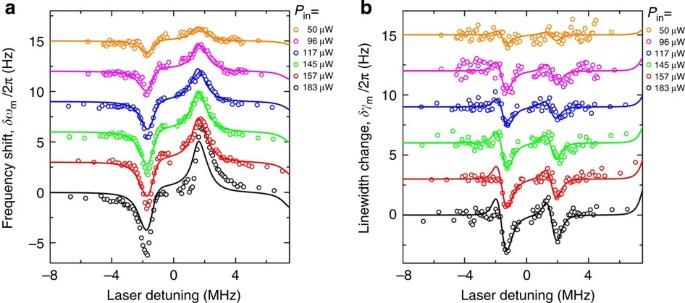Figure 3: Optomechanics at an avoided crossing. (a–b) Changes in the frequency (a) and linewidth (b) of the membrane’s fundamental mode as a function of the control laser detuning Δ and control beam powerPin. The membrane is nominally at the avoided crossing (zdis=0 nm).Pinandzdisare the fit parameters for the theory curves. The fit results forPinare shown in the legend. The fit results forzdishad a mean value of 0.32 nm with a s.d. of 0.03 nm. For clarity, each curve is shifted vertically by 3 Hz. Figure 3 shows similar measurements, but carried out at fixed z dis ≈0 nm as a function of the control beam power P in . The data are plotted along with the predictions of the model. These predictions use the parameter values taken from the fits in Fig. 2 , except for z dis and P in , which are used as fit parameters (the fit values of z dis and P in agree well with independent measurements, as described in the Supplementary Fig. 7 ). Figure 3 shows clearly that when z dis ≈0 nm, the feature in δ ω m has an even symmetry at each cavity resonance while the feature in δ γ m has odd symmetry, in agreement with theory. Figure 3: Optomechanics at an avoided crossing. ( a – b ) Changes in the frequency ( a ) and linewidth ( b ) of the membrane’s fundamental mode as a function of the control laser detuning Δ and control beam power P in . The membrane is nominally at the avoided crossing ( z dis =0 nm). P in and z dis are the fit parameters for the theory curves. The fit results for P in are shown in the legend. The fit results for z dis had a mean value of 0.32 nm with a s.d. of 0.03 nm. For clarity, each curve is shifted vertically by 3 Hz. Full size image Previous measurements of static reflection spectra at room temperature showed that it is possible to tune the avoided crossings by adjusting the membrane’s tilt relative to the cavity axis, and its position along the cavity axis [29] , [32] (see also ref. 35 ). To illustrate this capability at T =500 mK and to demonstrate its impact on the optomechanical dynamics, cavity spectra are shown in Fig. 4a,b for two different membrane alignments. When the membrane is positioned near the cavity waist with nominally zero tilt ( Fig. 4a ), only one of the triplet modes forms an avoided crossing with the singlet mode. After translating the membrane by −15 μm along the cavity axis and tilting it by 0.3 mrad ( Fig. 4b ), two of the triplet modes form avoided crossings. 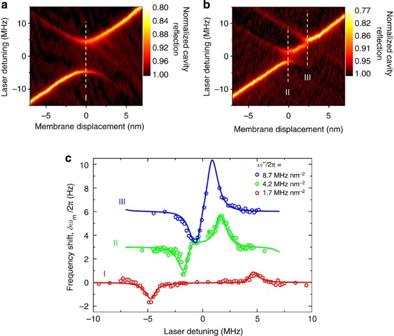Figure 4: Optomechanics as the avoided crossings are tuned. (a–b) Cavity reflection spectrum for two different membrane alignments: membrane located at the cavity waist with a tilt of ~0 mrad (a) and translated −15 μm along the cavity axis and tilted 0.3 mrad (b). The data in (b) is reproduced fromFig. 1d. The three avoided crossings have quadratic coefficients(I), 4.2 MHz nm−2(II) and 8.7 MHz nm−2(III). (c) The membrane’s frequency shift measured at the three avoided crossings as a function of the control laser detuning. For each measurement,Pin=80 μW. For clarity, each curve is shifted vertically by 3 Hz. SeeSupplementary Informationfor details of the theory and fit results. The data inFigs 2and3were measured using the crossing with. Figure 4: Optomechanics as the avoided crossings are tuned. ( a – b ) Cavity reflection spectrum for two different membrane alignments: membrane located at the cavity waist with a tilt of ~0 mrad ( a ) and translated −15 μm along the cavity axis and tilted 0.3 mrad ( b ). The data in ( b ) is reproduced from Fig. 1d . The three avoided crossings have quadratic coefficients ( I ), 4.2 MHz nm −2 ( II ) and 8.7 MHz nm −2 ( III ). ( c ) The membrane’s frequency shift measured at the three avoided crossings as a function of the control laser detuning. For each measurement, P in =80 μW. For clarity, each curve is shifted vertically by 3 Hz. See Supplementary Information for details of the theory and fit results. The data in Figs 2 and 3 were measured using the crossing with . Full size image Figure 4c shows measurements of δ ω m (Δ) for each of the three avoided crossings in Fig. 4a,b . For each measurement, z dis was set so that the membrane was at the avoided crossing. The solid lines are fits to the same model as the previous figures. As the avoided crossing gap is decreased, the peaks in δ ω m move close together and grow larger, reflecting the increase in . For the uppermost trace, the gap at the avoided crossing is no longer substantially larger than κ , and the two peaks begin to merge. See Supplementary Table S2 for a full description of the fit results. Classical analogue of a quantum non-demolition measurement Proposals for realizing a quantum non-demolition measurement of the membrane’s phonon number or the cavity’s photon number make use of the fact that at an avoided crossing, a change in the number of quanta in one oscillator (optical or mechanical) shifts the frequency of the other oscillator by g 2 . Detecting individual quantum jumps with such a measurement requires single-quantum strong coupling [30] , which has not been achieved in optomechanical devices to date. However, even without single-quantum strong coupling the non-demolition nature of these measurements is predicted to enable the detection of non-classical fluctuations of a driven oscillator [15] , [16] . Here we demonstrate a classical analogue of such a measurement by using the membrane’s resonance frequency ω m to monitor classical fluctuations of the intracavity laser power. These fluctuations are produced by modulating the power of the control laser with a frequency 75 Hz and depth 0.77. At the same time, the membrane’s fundamental mode is driven (using the piezo element) in a phase-locked loop (PLL). The PLL ensures that the frequency of the piezo drive tracks fluctuations in ω m and the PLL error signal provides a record of these fluctuations (see the Supplementary Methods for details). 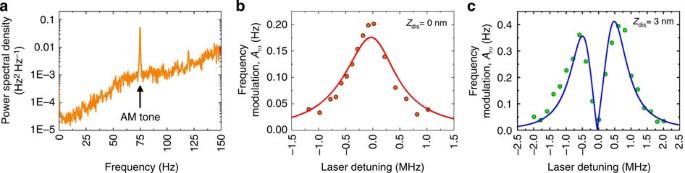Figure 5: Observing laser fluctuations via quadratic optomechanics. (a) Spectrum of the membrane’s resonance frequency,Sffmeasured using a PLL. The sharp peak at 75 Hz results from the intensity modulation (modulation depthβ=0.77) applied to the control beam, which modulates the membrane’s frequency via the quadratic optomechanical coupling. (b,c) The amplitude of the peak inSff, plotted versus control laser detuning atzdis=0 nm (b) andzdis=3 nm (c). The solid lines are fit to the absolute value of the expected optical spring. The fit results arezdis=−0.14±0.07 nm,β=0.67±0.15 forbandzdis=3.09±0.01 nm,β=0.67±0.14 forc. The quoted errors are statistical fit errors. The data in this figure was taken using the lower branch of the avoided crossing ‘I’ inFig. 4a. Figure 5a shows S ff , the spectrum of these fluctuations, when the membrane is positioned at an avoided crossing ( z dis =0 nm in Fig. 4a ) and the control beam is tuned to the cavity resonance (Δ=0). The peak in S ff at 75 Hz reflects the response of ω m to the laser’s modulation. Figure 5: Observing laser fluctuations via quadratic optomechanics. ( a ) Spectrum of the membrane’s resonance frequency, S ff measured using a PLL. The sharp peak at 75 Hz results from the intensity modulation (modulation depth β =0.77) applied to the control beam, which modulates the membrane’s frequency via the quadratic optomechanical coupling. ( b , c ) The amplitude of the peak in S ff , plotted versus control laser detuning at z dis =0 nm ( b ) and z dis =3 nm ( c ). The solid lines are fit to the absolute value of the expected optical spring. The fit results are z dis =−0.14±0.07 nm, β =0.67±0.15 for b and z dis =3.09±0.01 nm, β =0.67±0.14 for c . The quoted errors are statistical fit errors. The data in this figure was taken using the lower branch of the avoided crossing ‘I’ in Fig. 4a . Full size image Figure 5b and c shows A ω , the amplitude of the 75 Hz modulation of ω m as a function of Δ. In Fig. 5b , A ω (Δ) is measured with z dis =0 nm (that is, at an avoided crossing). The maximum value of A ω occurs at Δ=0, as expected for quadratic coupling. In contrast Fig. 5c , shows A ω (Δ) measured with z dis =3 nm (that is, far from an avoided crossing). In this case, A ω has a minimum at Δ=0 as expected for the linear coupling. The solid lines in Fig. 5b,c are fits to the same model as in the other figures. We emphasize that the important difference between the quadratic and linear coupling is not the specific form of A ω (Δ) (although measuring A ω (Δ) does provide a simple practical means for distinguishing them), but rather the different physical mechanisms by which the two couplings produce an optical spring. Specifically, the optical spring associated with linear coupling in single-mode devices arises from the leakage of light into and out of the cavity with each oscillation of the membrane [1] . In contrast, the optical spring associated with quadratic coupling results from the elastic energy stored in the intracavity field [34] . This distinction underlies a number of the proposed applications of these avoided crossings [15] , [16] , [17] , [18] . In summary, we have measured the dynamics of an optomechanical device in which multiple cavity modes are coupled by the motion of a single mechanical oscillator (in contrast with previous work, which has focused on static spectroscopy). We find that the avoided crossings between the cavity modes result in an optical spring that differs substantially from conventional, single-mode optomechanical devices. These results are in quantitative agreement with a classical theory of the device’s linear dynamics. This agreement, along with the demonstration of this device’s in situ tunability and cryogenic operation, are important steps towards studying the nonlinear and quantum regimes of multimode optomechanical devices. In particular, by improving this device’s cavity finesse and mechanical quality factor (as demonstrated in ref. 14 ), it should be possible to exploit multimode effects to efficiently produce squeezed states of the mechanical oscillator and optical field [19] , [20] , [21] , transfer states between cavity modes [17] , initialize macroscopic matter-wave interferometers [18] and measure the quantum statistics of a driven mechanical oscillator [15] , [16] . Following the description in ref. 42 , we represent the cavity field as a superposition of basis modes, which we take to be the cavity’s eigenmodes when the membrane is far from the avoided crossings. The amplitudes of these modes, a n , are the cavity’s degrees of freedom. The membrane couples these modes and detunes them by an amount that depends upon z dis and z osc (here z dis is the uniform translation of the membrane chip and z osc is the instantaneous displacement associated with the membrane’s oscillatory motion). For the small range of motion considered here, we assume that this detuning is linear in both z dis and z osc . These effects can be incorporated into the usual optomechanical equation of motion via the Hamiltonian , where the components of the vector are the mode amplitudes a n , b is the amplitude of the mechanical oscillation and M is a matrix whose diagonal elements represent the detuning of the cavity modes and whose off-diagonal terms represent the coupling between modes [42] . The optomechanical effects associated with the avoided crossings emerge from this model even in the simple case of just two optical modes ( n =1, 2); in this case This model allows the detuning associated with z dis to have different coefficients from the detuning associated with , since the exact location of the cavity mode on the membrane is not known a priori . The cavity spectra in Fig. 1b–d correspond to the case where z dis is varied (by scanning the voltage on a small piezoelectric element) while z osc =0 nm. In this case, the two cavity modes would cross at z dis =0 nm, but instead the off-diagonal terms in M produce a gap with magnitude 2 t . The Supplementary Note 1 provides a more detailed description of this model and describes how it is used to calculate the optical spring, optical damping and the cavity reflection spectrum. We note that although the restriction to two optical modes (equation (1)) provides an intuitive explanation of most of our data, we use three optical modes ( n =1, 2, 3) for most of the quantitative analysis. Explicit expressions for three optical modes are given in the Supplementary Note 1 ; they are straightforward extensions of equation (1) in which M includes two coupling terms ( and ) corresponding to the two avoided crossings seen in Fig. 1d . In fitting the cavity spectrum to this model (as in Fig. 1e ) there are a large number of fitting parameters; however the fits are highly constrained by the fact that each of the model’s parameters corresponds to a prominent feature in the data. For example, the three are set by the slopes of the cavity resonances far from the crossings, while the coupling rates t 1 and t 2 are determined by the magnitudes of the gaps. The coupling phases φ 1 and φ 2 are determined by the amplitudes of the cavity resonances near the crossing. Each mode’s κ is determined by the width of the resonance far from the crossing, while the input coupling of each mode is determined by the amplitude of the resonance far from the crossing. This analysis of the cavity’s static spectrum provides all the model parameters except for the three coefficients . The are extracted from fitting the optical spring and optical damping data in Fig. 2 , as described in the main body of the paper. How to cite this article: Lee, D. et al . Multimode optomechanical dynamics in a cavity with avoided crossings. Nat. Commun. 6:6232 doi: 10.1038/ncomms7232 (2015).